Whole exome sequencing of insulinoma reveals recurrent T372R mutations inYY1 Functional pancreatic neuroendocrine tumours (PNETs) are mainly represented by insulinoma, which secrete insulin independent of glucose and cause hypoglycaemia. The major genetic alterations in sporadic insulinomas are still unknown. Here we identify recurrent somatic T372R mutations in YY1 by whole exome sequencing of 10 sporadic insulinomas. Further screening in 103 additional insulinomas reveals this hotspot mutation in 30% (34/113) of all tumours. T372R mutation alters the expression of YY1 target genes in insulinomas. Clinically, the T372R mutation is associated with the later onset of tumours. Genotyping of YY1 , a target of mTOR inhibitors, may contribute to medical treatment of insulinomas. Our findings highlight the importance of YY1 in pancreatic β-cells and may provide therapeutic targets for PNETs. Pancreatic neuroendocrine tumours (PNETs) are classified into functional and non-functional tumours by hormone secretion and clinical symptoms. The main type of functional PNETs is insulinoma, which is derived from pancreatic β-cells and constantly secretes insulin or proinsulin. Germline mutations of MEN1 gene, which cause multiple endocrine neoplasia type 1, can lead to the development of insulinoma [1] . A recent study discovered frequent somatic mutations in MEN1 , DAXX/ATRX , TSC2 and PTEN genes in non-functional PNETs [2] . However, the major genetic basis of functional PNETs and the differences between functional and non-functional PNETs have not been fully elucidated. Genetic investigation of insulinoma may contribute to discovery of crucial genes controlling tumorigenesis, proliferation and functions of pancreatic β-cells. Moreover, previous studies have linked PNETs and diabetes studies via several key genes and pathways in pancreatic β-cells. The critical genes mutated in PNETs could be responsible for the physiological regulation of pancreatic β-cells. For example, MEN1 regulates compensatory proliferation of β-cells and promotes gestational diabetes in pregnant mice [3] . MEN1 could be targeted for reversing hyperglycaemia in diabetic mice [4] . The regulation of mammalian target of rapamycin (mTOR) pathway is crucial for both PNETs and diabetes [2] , [5] , [6] , [7] . Therefore, the further genetic explorations of insulinomas might provide potential therapeutic targets for both PNETs and diabetes. Here we identify recurrent T372R mutations in the transcription factor YY1 (Yin Yang 1) by whole exome sequencing, and validate this hotspot mutations in 30% sporadic insulinomas. Our results may contribute to a new diagnostic classification and medical therapy of PNETs. Recurrent YY1 T372R mutations in insulinomas To determine whether functional and non-functional PNETs share the similar driver genes, we screened mutations of MEN1 and DAXX/ATRX in 39 pairs of insulinoma and matched blood DNA. Compared with non-functional PNETs with 43% MEN1 and 44% DAXX / ATRX mutations, we only found one somatic mutation in MEN1 (2.5%) and one mutation in ATRX (2.5%). Global messenger RNA profiling of insulinomas and non-functional PNETs also showed distinctive expression patterns [5] . To explore the unique driver genes in sporadic insulinoma, 10 pairs of tumour and matched blood DNA excluding MEN1 and DAXX / ATRX mutations were selected for whole exome sequencing in discovery cohort ( Supplementary Table S1 ). Sequencing was performed on Hiseq2000 platform with NimbleGen 44M human exome array. The average sequencing depth was 157-fold (93X–200X), and 97.96% (97.50–98.60%) of the target regions were covered at least 10-fold ( Supplementary Table S2 and Supplementary Fig. S1 ). We identified 78 somatic mutations among the 10 tumours, including 21 synonymous, 49 missense, 1 nonsense, 3 splice sites and 4 frameshift ( Supplementary Table S3 ), resulting in an average of 8 (2–18) somatic mutations per tumour ( Supplementary Table S4 ). The most common substitution in these samples was the C:G>T:A transition, similar to most cancer types ( Supplementary Table S5 and Supplementary Fig. S2 ). Strikingly, YY1 harboured recurrent c.C1115G/p.T372R in three tumours, significantly higher ( P =5.4E−10, Poisson probability function [8] ) than the background. 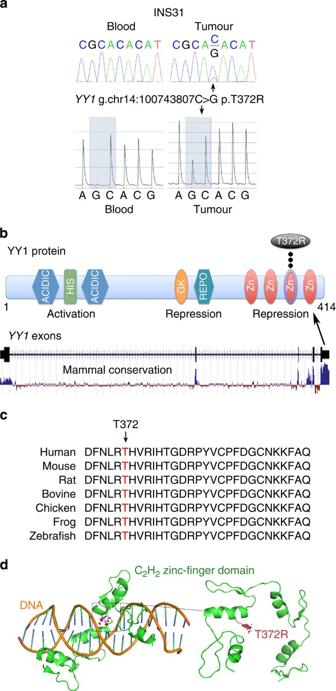Figure 1: Hotspot T372R mutations inYY1. (a) Validation of T372R mutation by Sanger sequencing and pyrosequencing. (b) Human YY1 protein and exons. Domains and motifs responsible for transcriptional regulation are indicated. Acidic, 11 consecutive acidic amino acids; His, histidine-rich domain; GK, glycine–lysine-rich domain; REPO, recruitment of polycomb domain; Zn, zinc-finger domain. Recurrent T372R mutations locate in the third zinc finger. (c) Conservation of T372 in zinc-finger domain. (d) Location of T372R mutation on crystal structure of C2H2-zinc-finger domain in YY1. In addition, we found somatic mutations in three potential cancer-related genes, including MLL3 , H3F3A and LMO2 ( Table 1 ). T372R mutation in YY1 has never been reported in publically available databases (including 1,000 genomes and dbSNP database). Table 1 Recurrent YY1 T372R mutations and mutated potential tumour-related genes in insulinomas. Full size table We validated the T372R mutations in YY1 , and then screened this mutation in 103 additional insulinomas by Sanger sequencing or pyrosequencing ( Fig. 1a and Supplementary Fig. S3 ). The screening cohort included matched tumour and blood DNA from frozen samples, and formalin-fixed and paraffin-embedded (FFPE) tumour tissues with partial-matched blood ( Supplementary Table S6 ). Our data showed that somatic c.C1115G/p.T372R mutation in YY1 existed in 30% sporadic insulinomas, including malignant (1/7) ones ( Supplementary Table S7 ). Figure 1: Hotspot T372R mutations in YY1 . ( a ) Validation of T372R mutation by Sanger sequencing and pyrosequencing. ( b ) Human YY1 protein and exons. Domains and motifs responsible for transcriptional regulation are indicated. Acidic, 11 consecutive acidic amino acids; His, histidine-rich domain; GK, glycine–lysine-rich domain; REPO, recruitment of polycomb domain; Zn, zinc-finger domain. Recurrent T372R mutations locate in the third zinc finger. ( c ) Conservation of T372 in zinc-finger domain. ( d ) Location of T372R mutation on crystal structure of C 2 H 2 -zinc-finger domain in YY1. Full size image Clinical features of YY1 T372R mutation in insulinomas To study the clinical significance of YY1 mutations, all patients in the cohort were divided into wild-type and T372R subgroups. The appearance of insulinomas with wild-type YY1 was significantly earlier than T372R subgroup in both male and female patients. 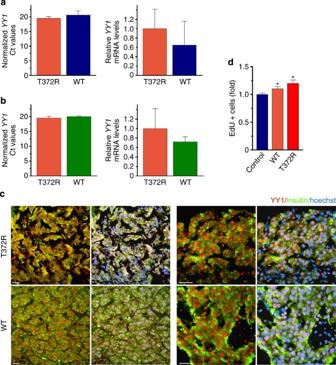Figure 2: Functional YY1 T372R mutations in insulinomas. (a) Quantitative reverse transcriptase (qRT)–PCR analysis of WT and T372R-mutatedYY1expression in insulinomas. Original Ct values were normalized to housekeeping geneGAPDH(WT group,n=8; T372R group,n=5). (b) qRT–PCR analysis of WT and T372R-mutatedYY1expression in normal human islets and insulinomas. Original Ct values were normalized to housekeeping geneGAPDH(T372R group,n=5; control group,n=3). All of samples are benign insulinomas. Data represent mean±s.d. (c) Insulinoma sections were stained with YY1 antibody (red) and insulin antibody (green). The data represents samples from six benign insulinomas in each group. Scale bars, 30 μm. (d) EdU staining and flow cytometric analysis. MIN6 cells were transfected with wild-type, T372R-mutated YY1 and vector control. The fold change of EdU-positive cells were analysed. Data represent mean ± SD, *P<0.05, Student's t-test. The data shown represents three independent experiments. There was no significant difference in the percentage of YY1 -mutated tumours between benign and malignant insulinomas in the cohort ( Table 2 and Supplementary Table S8 ). Quantitative analysis of Ki67 staining in insulinomas indicated similar proliferative activity between YY1 -mutated insulinoma cells and other tumour cells ( Supplementary Fig. S4 ). Interestingly, T372R mutation in YY1 was also reported in one adrenal aldosterone-producing adenoma [9] . In other cancers, including breast cancer, prostate cancer and colon cancer, overexpression of YY1 could be correlated with tumorigenesis and poor prognosis [10] . Table 2 T372R mutation in YY1 is associated with late onset of insulinomas. Full size table Functional T372R mutation in the zinc-finger domain of YY1 YY1 is an important regulatory node in tumorigenesis, glucose metabolic homoeostasis and epigenetic regulation processes [11] , [12] , [13] , [14] , [15] . YY1 encodes a ubiquitously distributed transcription factor belonging to the GLI-Kruppel class of zinc-finger proteins. The highly conserved carboxy terminus C 2 H 2 -zinc-finger domains of YY1 are responsible for DNA binding and transcriptional repression. The repression domain of YY1 is mapped to the last two and a half zinc fingers (amino acid 333–amino acid 397) [12] . T372R mutation in YY1 locates in the third functional zinc-finger domain, indicating that it may affect the repression functions of YY1 ( Fig. 1b,c ). On the basis of co-crystal structure of protein–DNA binding between YY1 zinc fingers and AAV P5 initiator [16] , alterations in zinc-finger structure were predicted to locate on DNA-contacting surface, suggesting effects of T372R on DNA modifications and transcriptional regulation ( Fig. 1d ). Quantitative PCR analysis showed high YY1 expression in insulinomas with wild-type and mutated YY1 , as well as normal human islets. The expression levels of wild-type and mutated YY1 were not significantly changed in insulinomas ( Fig. 2a,b ). Immunofluorescence staining demonstrated that YY1 was mainly expressed in the nucleus of insulinoma cells ( Fig. 2c ). Further, in vitro 5-ethynyl-2′-deoxyuridine (EdU) proliferation assays indicate that overexpression of wild-type and mutated YY1 promotes proliferation of mouse insulinoma (MIN6) cells ( Fig. 2d ). Taken together, our results suggested that T372R in YY1 was a critical oncogenic mutation in insulinomas. Figure 2: Functional YY1 T372R mutations in insulinomas. ( a ) Quantitative reverse transcriptase (qRT)–PCR analysis of WT and T372R-mutated YY1 expression in insulinomas. Original Ct values were normalized to housekeeping gene GAPDH (WT group, n =8; T372R group, n =5). ( b ) qRT–PCR analysis of WT and T372R-mutated YY1 expression in normal human islets and insulinomas. Original Ct values were normalized to housekeeping gene GAPDH (T372R group, n =5; control group, n =3). All of samples are benign insulinomas. Data represent mean±s.d. ( c ) Insulinoma sections were stained with YY1 antibody (red) and insulin antibody (green). The data represents samples from six benign insulinomas in each group. Scale bars, 30 μm. ( d ) EdU staining and flow cytometric analysis. MIN6 cells were transfected with wild-type, T372R-mutated YY1 and vector control. The fold change of EdU-positive cells were analysed. Data represent mean ± SD, *P<0.05, Student's t-test. The data shown represents three independent experiments. Full size image T372R mutation increases the transcriptional activity of YY1 YY1 is a functional transcription factor in fundamental processes of cancer and metabolism [10] , [13] , [14] . Previous studies have demonstrated that YY1 is a common target of mTORC1. Inhibition of mTOR results in decreased mitochondrial function and insulin/insulin-like growth factor signalling by controlling YY1 activity in skeletal muscle [13] , [14] . mTOR inhibition can decrease the mitochondrial gene expression through direct modulation of YY1 activity, whereas overexpression of YY1 increases the expression of mitochondrial genes [13] . To explore T372R mutation-induced functional alterations of YY1, we examined the expression of a few YY1 target genes in insulinomas. Our data showed significantly increased expression of mitochondrial gene IDH3A and UCP2 in YY1 -mutated tumours. In addition, the expression of COL1A1 gene, which is positively regulated by YY1 (ref. 17 ), was significantly upregulated in YY1 -mutated tumours ( Fig. 3 ). These results suggested that T372R mutation could enhance the transcriptional activity of YY1. 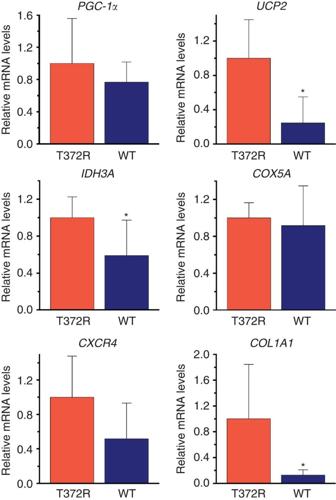Figure 3: Expression of YY1 target genes in insulinomas. qRT–PCR analysis ofPGC1α,UCP2,IDH3A,COX5A,CXCR4andCOL1A1expression was performed (n=6 for each group). All of samples are benign insulinomas. Data represent mean±s.d., *P<0.05, Student’st-test. Figure 3: Expression of YY1 target genes in insulinomas. qRT–PCR analysis of PGC1α , UCP2 , IDH3A , COX5A , CXCR4 and COL1A1 expression was performed ( n =6 for each group). All of samples are benign insulinomas. Data represent mean±s.d., * P <0.05, Student’s t -test. Full size image YY1 regulates the mitochondrial function and insulin/insulin-like growth factor signalling, which is crucial for pancreatic β-cell survival and insulin secretion [13] , [14] , [18] , [19] . Our data indicate that T372R mutation enhances the transcriptional activity of YY1. Overexpression of mutated and wild-type YY1 promotes proliferation of MIN6 cells. T372R mutation in YY1 and overexpression of wild-type YY1 might have similar effects. These studies have shed light on the importance of YY1 in energy metabolism. The precise functions of YY1 in pancreatic β-cells could be investigated in transgenic mouse models and human islets in the future. The comprehensive understanding of physiological and pathological functions of YY1 in β-cells might provide potential therapeutic targets for diabetes. Recently, the medical therapy of insulinoma and PNETs has been investigated in a series of clinical studies [20] , [21] . Everolimus (RAD001), an oral mTOR inhibitor, substantially improves glycaemic control and reduces the tumour size in patients with insulinoma [20] . Phase 2 and 3 clinical trials demonstrated that Everolimus could prolong progression-free survival in patients with advanced PNETs [21] . However, the molecular mechanisms underlying these significant therapeutic effects are still unclear. Interestingly, our results revealed a potentially activating YY1 mutation in 30% insulinomas, which might be treated with drugs targeting the activity of YY1. Consistently, the mTOR inhibitors can control and modify the transcriptional activity of YY1. Therefore, YY1 genotyping may contribute to diagnostic classification of insulinomas and improve mTOR inhibitors’ therapy in the future. Collectively, our study reveals the YY1 mutation hotspot T372R as an oncogenic mutation in 30% sporadic insulinomas. These findings may provide new diagnostic and therapeutic approaches for PNETs. Clinical samples Insulinomas were diagnosed by clinical hypoglycaemia symptoms, blood insulin and glucose levels (prolonged oral glucose tolerance test), computed tomography/positron emission tomography-computed tomography imaging of patients and pathological diagnosis of surgical removal tumour. Genomic DNA was obtained from matched frozen insulinoma tumour and blood samples, and FFPE insulinoma tissues with partial-matched blood in the endocrine-related tumour bank of Shanghai Key Laboratory for Endocrine Tumors. Only matched frozen samples were used in the discovery cohort. DNA was prepared with QIAGEN DNeasy Blood & Tissue Kit and QIAamp DNA FFPE Tissue Kit. Normal human pancreatic islets were isolated from the donor pancreas for transplantation. Normal human islets of Langerhans used in this study were isolated according to the Edmonton protocol. Total RNA was prepared with QIAGEN miRNeasy mini kit. Informed consent was obtained from all study participants. All the protocols were approved by the Rui-jin Hospital Ethics Committee, Shanghai Jiao Tong University School of Medicine. Exome sequencing The qualified genomic DNA from tumour and matched peripheral blood from 10 insulinomas were fragmented by Covaris technology with resultant library fragments 200–300 bp, and then adapters were ligated to both ends of the fragments. Extracted DNA was then amplified by ligation-mediated PCR, purified and hybridized to the NimbleGenEZ 44M human exome array for enrichment, non-hybridized fragments were then washed out. Both non-captured and captured ligation-mediated PCR products were subjected to quantitative PCR to estimate the magnitude of enrichment. Each captured library was then loaded on Hiseq2000 platform, and we performed high-throughput sequencing for each captured library independently to ensure that each sample meet the desired average fold-coverage. Raw image files were processed by Illumina base calling Software 1.7 for base calling with default parameters and the sequences of each individual were generated as 90 bp paired-end reads. Reads mapping and variation detection After removing reads containing sequencing adapters and low-quality reads with more than five unknown bases, high-quality reads were aligned to the NCBI human reference genome (hg19) using Burrows–Wheeler Aligner (v0.5.9) [22] with default parameters. Picard (v1.54) [23] was employed to mark duplicates and followed by Genome Analysis Toolkit (v1.0.6076, GATK IndelRealigner) [24] to improve alignment accuracy. Potential somatic single nucleotide variants were predicted by Varscan2.2.5 (with parameters as http://www.varscan.sourceforge.net/samtools (v0.1.18) [25] mpileup –Q 0 and Varscan2.2.5 --min-coverage 10 --min-coverage-normal 10 --min-coverage-tumour 10 --min-var-freq 0.1 --min-freq-for-hom 0.75 --min-avg-qual 0) [26] . Then we use our house pipeline to identify somatic mutations, with major criteria as the following: adjacent somatic mutation distance, mapping quality, base quality, allele frequency change between tumour and adjacent normal, mutation should not be in gap-aligned reads, mutations should not be significantly enriched within 5 bp of 5′- or 3′-ends of the reads and mutations should not be in simple repeat region. Somatic InDels were predicted by GATK SomaticIndelDetector with default parameters. Then we developed own pipeline to get high confidence somatic indels, as following: combined normal and tumour bam were reused to perform local realignment and germline indels were filtered for high confidently indels, normal coverage and tumour coverage should be ≥10. High confidently somatic single nucleotide variants and InDels were annotated using ANNOVAR (released 2011-10-02) [27] . Validation of YY1 mutation by PCR and Sanger sequencing PCR was performed on Dual 96-well GeneAmp PCR System 9700 (Applied Biosystems), 20 ng template DNA from each sample was used per reaction. The products were sequenced by 3730xl DNA Analyzer (Applied Biosystems). All sequences were analysed by the Sequencing Analysis Software Version 5.2 (Applied Biosystems). Following primers were used: 5′-CACCCAGGGCAGGAATG-3′ for human YY1 -F1; 5′-CCTGTCTCCGGTATGGA-3′ for human YY1 -R1. Validation of mutations by pyrosequencing Pyrosequencing was performed on QIAGEN PyroMark Q96 ID system with PyroMark Q96 Vacuum Workstation and PyroMark Gold Q96 Reagents, following the instructions in the user manual. Following primers were used: 5′-GGGAAACGCTTTTCACTGGAC-3′ for human YY1 -F2; 5′-TAGGGCCTGTCTCCGGTATG-3′ for human YY1 -R2 and 5′-GGTATGGATTCGCACA-3′ for sequencing. Immunofluorescence staining FFPE insulinoma tissues were deparaffinized using standard techniques. Immunofluorescence staining were performed according to the standard protocol. The following primary antibodies were used: polyclonal rabbit anti-YY1 antibody (1:100; ORIGENE, clone EPR4651) and polyclonal guinea pig anti-insulin (1:400; Dako). The secondary antibodies for immunofluorescence staining were purchased from Invitrogen and Dako. The images were acquired using an Olympus microscopy system. Real-time reverse transcription–PCR Total RNA was extracted using QIAGEN miRNeasy mini kit. For reverse transcription, 1 μg of total RNA was converted into first-strand complementary DNA in a 20-μl reaction volume using a reverse transcription kit following the manufacturer’s instruction. Quantitative real-time PCR was then performed using a LightCycler 480 Real-Time PCR System (Roche Applied Science). The comparative cycle threshold method was used to determine the relative messenger RNA expression of human YY1 after normalization to housekeeping gene GAPDH . The following primers were used: 5′-CCTGGCATTGACCTCTCAGATCCCA-3′ for human YY1 -F3; 5′-GGGCAAGCTATTGTTCTTGGAGCA-3′ for human YY1 -R3. 5′-TTTGCCATGAAGTTCAATGCA-3′ for human PGC1α -F, 5′-AGCAGCCACAAAAAGGGAGAT-3′ for human PGC1α -R. 5′-GGTTCCTGGAACGTGGTGAT-3′ for human Ucp2 -F, 5′-AGCCATGAGGGCTCGTTTC-3′ for human Ucp2 -R. 5′-TGCTGCCAAAGCACCTATTCA-3′ for human idh3a -F, 5′-GTGACCGGCTGCTATTGGG-3′ for human idh3a -R. 5′-TCGCCGTCATGCTGGG-3′ for human COX5a -F, 5′-CAATAAATCCTTGGGGAAGCC-3′ for human COX5a -R. 5′-GGAGGGGATCAGTATATACA-3′ for human CXCR4 -F, 5′-GAAGATGATGGAGTAGATGG-3′ for human CXCR4 -R. 5′-CACCAATCACCTGCGGTACAGAA-3′ for human Col1a1 -F, 5′-CAGATCACGTCATCGCACAAC-3′ for human Col1a1 -R. Cell culture and transfection Mouse MIN6 cell lines were kindly provided by Dr. Xiao Wang (Shanghai Institute of Endocrine and Metabolic Diseases) and cultured as described previously [28] , [29] . MIN6 cells were transfected with plasmids by Lipofectamine 2000 (Invitrogen). Human full-length YY1 complementary DNA was inserted in pCMV6 vector. T372R mutation was introduced into plasmids with the QuikChange II site-directed mutagenesis kit (Stratagene, La Jolla, CA) according to the manufacturer’s instruction. Flow cytometric analysis MIN6 cells were transfected with wild-type, T372R-mutated YY1 and vector controls for analysis. EdU staining was performed 24 h after transfection. Cell proliferation assay was performed using EdU assay kit (Click-iT EdU Flow Cytometry Assay Kit, Invitrogen); positive cells were analysed by flow cytometry. Computational modelling of T372R in YY1 The available protein crystal structures of Human YY1 residues 293–414 and crystallization DNA complex (PDB 1UBD) were identified as the template [16] . A three-dimensional model of the YY1 C 2 H 2 -zinc-finger domains and DNA complex and T372R mutation was generated using PyMOL software [30] . Statistical analysis Recurrent mutated YY1 was identified as a significant mutated gene as described before [8] . Significant differences were analysed using Student’s t -test or Fisher’s exact test. Error bars in graphs represent s.d. Differences were considered significant if P <0.05. Accession codes: The exome sequencing data has been deposited in the NCBI Sequence Read Archive database under the accession code SRA108014 . How to cite this article: Cao, Y. et al . Whole exome sequencing of insulinoma reveals recurrent T372R mutations in YY1. Nat. Commun. 4:2810 doi: 10.1038/ncomms3810 (2013).